Vertically grown ultrathin Bi2SiO5as high-κsingle-crystalline gate dielectric 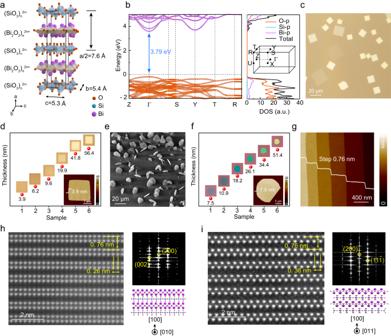Fig. 1: Structure, growth, and characterization of ultrathin Bi2SiO5single crystals. aCrystal structure of Bi2SiO5(Cc,a= 15.12 Å,b= 5.44 Å,c= 5.29 Å,β= 90.07°) with alternatively stacked [Bi2O2]n2n+and [SiO3]n2n−layers.bCalculated band structure and density of states (DOS) of Bi2SiO5with a direct band gap of ~3.79 eV. The first Brillouin zone is inserted in the right panel.cTypical optical micrograph (OM) image of square Bi2SiO5nanoplates showing an in-plane growth mode on mica substrate.dOM images of Bi2SiO5nanoplates with thickness-dependent color contrasts on mica. The inset shows the typical atomic force microscope (AFM) image of an ultrathin Bi2SiO5nanoplate with a thickness of 3.9 nm (5 layers) and an atomically smooth surface.eScanning electron microscopy (SEM) image of 2D Bi2SiO5crystals vertically grown on mica substrate.fThickness-dependent color contrasts for Bi2SiO5nanoplates transferred onto SiO2/Si substrate by a polymer-free mechanical pressing. The AFM image of a 7.5-nm-thick Bi2SiO5nanoplate was inserted inf.gTypical AFM image of a terraced Bi2SiO5nanoplates with a clear step of 0.76 nm.h,iCross-sectional atomic-resolved high angle annular dark field (HAADF) images (left) and corresponding fast Fourier transform (FFT) diffraction spots (right) of chemical vapor deposition (CVD) grown Bi2SiO5nanoplates taken along the zone axes of [010] (h) and [011] (i), respectively. Single-crystalline high- κ dielectric materials are desired for the development of future two-dimensional (2D) electronic devices. However, curent 2D gate insulators still face challenges, such as insufficient dielectric constant and difficult to obtain free-standing and transferrable ultrathin films. Here, we demonstrate that ultrathin Bi 2 SiO 5 crystals grown by chemical vapor deposition (CVD) can serve as excellent gate dielectric layers for 2D semiconductors, showing a high dielectric constant (>30) and large band gap (~3.8 eV). Unlike other 2D insulators synthesized via in-plane CVD on substrates, vertically grown Bi 2 SiO 5 can be easily transferred onto other substrates by polymer-free mechanical pressing, which greatly facilitates its ideal van der Waals integration with few-layer MoS 2 as high- κ dielectrics and screening layers. The Bi 2 SiO 5 gated MoS 2 field-effect transistors exhibit an ignorable hysteresis (~3 mV) and low drain induced barrier lowering (~5 mV/V). Our work suggests vertically grown Bi 2 SiO 5 nanoflakes as promising candidates to improve the performance of 2D electronic devices. Two-dimensional (2D) semiconductors hold great promise for fabricating more-than-Moore transistors and exploring the emergent transport properties [1] , [2] , [3] , [4] , [5] , but achieving their theoretical performance also requires compatible high- k dielectrics to guarantee efficient gate control [6] , [7] , [8] , [9] , [10] . Compared to traditional amorphous dielectrics (Al 2 O 3 and HfO 2 ) [11] , [12] , [13] , single-crystalline gate insulators with dangling-bond-free surfaces are more competitive to fabricate high-performance 2D devices with reduced interfacial scatterings and gate hysteresis [14] , [15] , [16] , [17] , [18] . For example, hexagonal boron nitride ( h -BN) has been widely used as a van der Waals (vdWs) substrate to improve carrier mobility and investigate exotic properties of 2D materials [19] , [20] , [21] , [22] , [23] . However, h -BN is also well known for its shortcomings of low dielectric constant ( k = 2~4) and harsh conditions (pressure: >4 G Pa, temperature: >1673 K) for the growth of high-quality single crystals [24] . Therefore, it is highly desirable to discover new vdWs insulators similar to h -BN, but has a much higher dielectric constant and more facile synthetic conditions, for exploring the emergent transport properties of 2D materials in a high- κ dielectric environment, as well as for fabricating 2D-material-based electronic devices with scaled supply voltage [15] , [16] . Even so, very rare have succeeded [18] , [25] . Very recently, Peng et al. [18] reported the synthesis of Bi 2 SeO 5 bulk crystals grown by chemical vapor transport (CVT), which can be exfoliated into few-nanometer-thick nanosheets and serve as an “ h -BN” like high- k dielectric to improve the mobility of 2D materials and enable the observation of quantum Hall effects in Bi 2 O 2 Se. Nevertheless, the CVT process for the synthesis of Bi 2 SeO 5 bulk crystals is also very time-consuming (typically ~40 days). Besides, similar to other vdWs dielectrics, transferable Bi 2 SeO 5 nanoflakes with suitable thicknesses and domain sizes were also prepared by a low-efficiency method of mechanical exfoliation for subsequent vdWs device integration. Compared to mechanical exfoliation, direct growth of free-standing ultrathin 2D insulators with high- k nature by chemical vapor deposition (CVD) is much more efficient, but remains challenging. Typically, CVD-grown atomically thin 2D insulators with a layered crystal structure preferably adopt an in-plane growth mode on substrates [26] , [27] , [28] , [29] , which will inevitably set obstacles for clean sample transfer and subsequent vdWs integration. However, if an ultrathin 2D insulator can be vertically grown on the substrate, just like the case in Bi 2 O 2 Se [3] , [30] , [31] , the transfer problem can be easily overcome due to much reduced interfacial interaction. Bi 2 SiO 5 is a well-known high- κ dielectrics with an Aurivillius-type layered structure and a large band gap of 3.5~4.4 eV [32] , [33] , [34] , [35] . According to the previous works regarding the bulk single crystals and polycrystalline powders of Bi 2 SiO 5 , Bi 2 SiO 5 shows an anisotropic dielectric constant [36] , [37] and its out-of-plane dielectric constant can be as high as 30~80 [36] , [37] , [38] , [39] , and thus was suggested as a potential candidate for high-temperature dielectrics [39] . Here, Bi 2 SiO 5 was demonstrated as an excellent gate dielectric for 2D semiconductors. Ultrathin Bi 2 SiO 5 single crystals with thickness down to monolayer were successfully synthesized by a facile CVD method, concurrently owing to the high dielectric constant (>30), large band gap (~3.8 eV), and large breakdown field strength. Remarkably, the preferable CVD growth mode of Bi 2 SiO 5 can be regulated from in-plane to out-of-plane under optimized conditions, showing great feasibility on sample transfer by polymer-free mechanical pressing. Using ultrathin Bi 2 SiO 5 nanoflakes as the vdW dielectrics and screening layers, we can greatly regulate the carrier density and improve the carrier mobility of few-layer MoS 2 (almost fifteen times higher than on the SiO 2 substrate at 5 K). Besides, the MoS 2 field-effect transistors (FETs) using Bi 2 SiO 5 as dielectrics can operate at 0.5 V, exhibiting a large I on / I off (>10 8 ), an ignorable hysteresis (~3 mV), low DIBL value (~5 mV/V) and low gate leakage current (~10 −13 A). Structure, CVD growth, and characterization of layered Bi 2 SiO 5 As shown in Fig. 1a , bismuth silicate Bi 2 SiO 5 possesses a monoclinic lattice with Cc space group (quasi-orthogonal, a = 15.12 Å, b = 5.44 Å, c = 5.29 Å, β = 90.07°) and has an Aurivillius-type layered crystal structure with alternatively stacked [Bi 2 O 2 ] n 2n+ and [SiO 3 ] n 2n- layers along the a -axis. The first-principle calculations were performed to investigate the band structure of layered Bi 2 SiO 5 . As shown in Fig. 1b , Bi 2 SiO 5 exhibits a large direct band gap of ~3.79 eV, whose conduction band minimum (CBM) and valance band maximum (VBM) are both locate at Γ point of the first Brillouin zone and mainly originate from Bi- p and O- p orbits, respectively. Fig. 1: Structure, growth, and characterization of ultrathin Bi 2 SiO 5 single crystals. 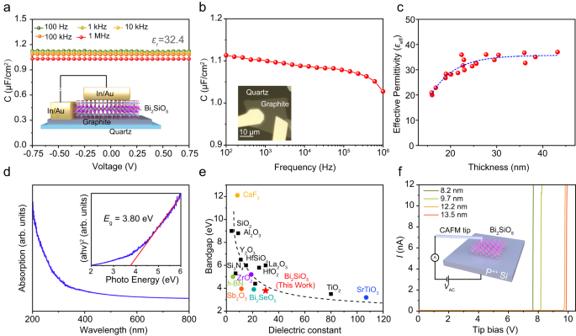Fig. 2: Dielectric constant, band gap, and breakdown field strength of CVD-grown Bi2SiO5nanoflakes. aTypical Bias-dependent capacitance (C) measurements on CVD-grown Bi2SiO5nanoflake with a common metal-insulator-metal (MIM) device configuration, where the thick graphite and In/Au metals serve as the bottom and top electrodes (inset), respectively. The dielectric constant (ɛr) of Bi2SiO5was estimated as ~32.4 at 100 Hz.bCorresponding frequency-dependent capacitance (C–f) characteristics of the MIM device, whose OM image is inset inb.cThe thickness-dependent effective permittivity (εeff) of Bi2SiO5nanoflakes with a measuring frequency of 100 Hz. The dashed blue curve is a visual guide.dUltraviolet-visible (UV-vis) absorption spectrum of CVD-grown Bi2SiO5nanoflakes transferred onto quartz substrate with high coverage by mechanical pressing. The inset shows the fitting of its optical band gap (~3.8 eV) by Tauc’s law, wherea,h,andνare the absorption coefficient, Planck constant and frequency, respectively.eEnergy band gap versus dielectric constant of representative dielectric materials in literature, showing the coexistence of high dielectric constant and large band gap in Bi2SiO5. The dashed line is a visual guide.fThickness-dependent current-voltage curves of Bi2SiO5nanoplates measured by C-AFM, showing a high breakdown field strength of 9.4 MV/cm (8.2 nm). a Crystal structure of Bi 2 SiO 5 ( Cc , a = 15.12 Å, b = 5.44 Å, c = 5.29 Å, β = 90.07°) with alternatively stacked [Bi 2 O 2 ] n 2n+ and [SiO 3 ] n 2n− layers. b Calculated band structure and density of states (DOS) of Bi 2 SiO 5 with a direct band gap of ~3.79 eV. The first Brillouin zone is inserted in the right panel. c Typical optical micrograph (OM) image of square Bi 2 SiO 5 nanoplates showing an in-plane growth mode on mica substrate. d OM images of Bi 2 SiO 5 nanoplates with thickness-dependent color contrasts on mica. The inset shows the typical atomic force microscope (AFM) image of an ultrathin Bi 2 SiO 5 nanoplate with a thickness of 3.9 nm (5 layers) and an atomically smooth surface. e Scanning electron microscopy (SEM) image of 2D Bi 2 SiO 5 crystals vertically grown on mica substrate. f Thickness-dependent color contrasts for Bi 2 SiO 5 nanoplates transferred onto SiO 2 /Si substrate by a polymer-free mechanical pressing. The AFM image of a 7.5-nm-thick Bi 2 SiO 5 nanoplate was inserted in f . g Typical AFM image of a terraced Bi 2 SiO 5 nanoplates with a clear step of 0.76 nm. h , i Cross-sectional atomic-resolved high angle annular dark field (HAADF) images (left) and corresponding fast Fourier transform (FFT) diffraction spots (right) of chemical vapor deposition (CVD) grown Bi 2 SiO 5 nanoplates taken along the zone axes of [010] ( h ) and [011] ( i ), respectively. Full size image The essential prerequisite for using Bi 2 SiO 5 as single-crystalline dielectrics with strong gate control is to achieve its growth of atomically thin films. However, the CVD growth of ultrathin Bi 2 SiO 5 crystals remains a challenge yet. To our knowledge, SiO 2 is chemically inert and has a very high melting point, which prevents it to be used as Si supplier during the CVD growth of Si-based compounds to some extent. Nevertheless, it’s well known that the fluorides will react with SiO 2 to form volatile Si-based precursors. As a result, we developed a facile CVD method for the synthesis of Bi 2 SiO 5 ultrathin crystals by using the BiF 3 powders as Bi supplier and SiO 2 powders or quartz boat as Si supplier (see Supplementary Fig. 1 ). With this method, ultrathin Bi 2 SiO 5 crystals with various thicknesses can be readily obtained on mica substrates. As shown in Fig. 1c, d and Supplementary Fig. 2 , at a relatively high growth temperature (~1023 K), Bi 2 SiO 5 adopts a preferable in-plane growth mode on mica, which is widely observed in the CVD synthesis of layered materials, revealing a transparent square-like shape and atomically thin nature (down to monolayer, Supplementary Fig. 3 ). Normally, the in-plane growth mode will result in a large attaching area and strong bonding force between the epitaxial layer and the substrate, thereby adding difficulties for sample transfer and subsequent vdWs integration. Remarkably, the preferable growth mode of Bi 2 SiO 5 on mica can be regulated from in-plane to out-of-plane growth modes just by lowering its growth temperature, which is similar to the case of Bi 2 O 2 Se [30] . As shown in Fig. 1e and Supplementary Fig. 2b, c , vertically grown ultrathin Bi 2 SiO 5 crystals gradually emerge on mica at ~973 K, then dominates the CVD growth while further lowering the temperature to ~923 K. Unlike the case in Fig. 1c , vertically grown Bi 2 SiO 5 crystals with thickness ranging from 7.5 to 50 nm can be easily transferred onto various substrates (such as SiO 2 /Si, Fig. 1e ) by a polymer-free mechanical pressing (Supplementary Fig. 4 ), showing an atomically flat surface even after sample transfer (Fig. 1f ). The transferable feature without unfavorable residual polymer contaminations makes free-standing Bi 2 SiO 5 appealing for fabricating vdWs heterojunction device. Occasionally, the CVD-grown Bi 2 SiO 5 nanoflakes revealed a terraced morphology with a step height of ~0.76 nm (Fig. 1g ), consistent with the theoretical value for the monolayer step in Bi 2 SiO 5 . It’s worth noting that the CVD-grown Bi 2 SiO 5 shows excellent air stability, whose surface morphology and roughness of Bi 2 SiO 5 nanoplates remain almost the same when exposed to air for more than 7 months, which is an important metric for device fabrication as a high- κ gate dielectric (Supplementary Figs. 5 , 6 ). More details about the comparison experiments conducted to understand how the reaction goes in the CVD growth of Bi 2 SiO 5 and the possible reason for its in-plane and out-of-plane growth can be found in the discussion part of supporting information (Supplementary Figs. 7 , 8 ). The crystalline phase of as-grown samples was confirmed by transmission electron microscopy (TEM), Raman spectroscopy, and X-ray diffraction (XRD). As shown in Fig. 1h, i and Supplementary Fig. 9 , we performed high-resolution TEM imaging along three-zone axes [namely (010), (011), and (100)], as well as corresponding fast Fourier transform (FFT) fringes. Based on the atomic-resolved cross-sectional TEM technique, the alternative stacking of [Bi 2 O 2 ] n 2n+ and the [SiO 3 ] n 2n− layers with a layer space of 0.76 nm was observed. Besides, the averaged atomic ratio of Bi/Si was measured close to 2: 1 by energy dispersive spectroscopy (EDS, Supplementary Figs. 9 , 10 ), which is consistent with the chemical formula of Bi 2 SiO 5 . The active modes at 70, 97, 149, 208, 298, 372, 433 cm −1 of the Raman spectra also matched well with monoclinic Cc phase of Bi 2 SiO 5 (Supplementary Fig. 11 ) [35] . Additionally, the sharp XRD peaks, which can be assigned to ( h 00) crystal planes, further confirmed the high crystalline quality of the CVD-grown Bi 2 SiO 5 nanoplates (Supplementary Fig. 11c ). Dielectric properties of vertically grown Bi 2 SiO 5 nanoplates The transfer feasibility for vertically grown Bi 2 SiO 5 nanoplates greatly facilitates the evaluation of their intrinsic properties, such as dielectric constant, band gap, and breakdown field strength. As shown in Fig. 2a , metal-insulator-metal (MIM) capacitors were fabricated on quartz substrates to extract the dielectric constant of Bi 2 SiO 5 nanoflakes with varied thicknesses by capacitance-voltage ( C – V ) measurements. Here, the thick graphite and In/Au metals serve as the bottom and top electrodes, respectively. Thanks to high- κ nature, Bi 2 SiO 5 nanoflake with a thickness of 25.6 nm demonstrated a very high capacitance density of 1.12 μF/cm 2 at 100 Hz (Fig. 2a ), revealing a slight decrease when the measuring frequency is up to 1 MHz. The corresponding capacitance-frequency ( C – f ) measurements showed the similar results (Fig. 2b ). It is worth noting that the absolute capacitance value (>1 × 10 −12 F) measured is ~2~3 orders higher than the instrument’s offset and noise level (<1.5 × 10 −14 F, Supplementary Fig. 12 ). Based on the C – V and C – f data, we can estimate the effective permittivity ( ɛ eff ) of Bi 2 SiO 5 to be ~32.4 at 100 Hz, which is preferable than commercial amorphous high- κ oxide such as Al 2 O 3 ( k = 7~9) [13] , [40] , [41] and HfO 2 ( k = 13~17) [41] , [42] , and higher than most of reported vdWs single-crystalline dielectrics, such as h -BN ( k = ~3.5) [43] , [44] , CaF 2 ( k = 8.4) [14] , Bi 2 SeO 5 ( k = 15.6) [18] , VOCl ( k = 11.7) [45] and ZrO 2 ( k = 8~19) [17] . Furthermore, we investigated the thickness-dependent ɛ eff by fabricating MIM capacitors with different Bi 2 SiO 5 thicknesses, from which we can extract very large ɛ eff values of >30 in a wide thickness range (Fig. 2c ). The gradual decrease of ɛ eff while thinning down can be ascribed to the existence of interfacial “dead layer” in the MIM device, which is similar to other MIM devices [15] , [46] , [47] , [48] . Fig. 2: Dielectric constant, band gap, and breakdown field strength of CVD-grown Bi 2 SiO 5 nanoflakes. a Typical Bias-dependent capacitance ( C ) measurements on CVD-grown Bi 2 SiO 5 nanoflake with a common metal-insulator-metal (MIM) device configuration, where the thick graphite and In/Au metals serve as the bottom and top electrodes (inset), respectively. The dielectric constant ( ɛ r ) of Bi 2 SiO 5 was estimated as ~32.4 at 100 Hz. b Corresponding frequency-dependent capacitance ( C – f ) characteristics of the MIM device, whose OM image is inset in b . c The thickness-dependent effective permittivity ( ε eff ) of Bi 2 SiO 5 nanoflakes with a measuring frequency of 100 Hz. The dashed blue curve is a visual guide. d Ultraviolet-visible (UV-vis) absorption spectrum of CVD-grown Bi 2 SiO 5 nanoflakes transferred onto quartz substrate with high coverage by mechanical pressing. The inset shows the fitting of its optical band gap (~3.8 eV) by Tauc’s law, where a , h, and ν are the absorption coefficient, Planck constant and frequency, respectively. e Energy band gap versus dielectric constant of representative dielectric materials in literature, showing the coexistence of high dielectric constant and large band gap in Bi 2 SiO 5 . The dashed line is a visual guide. f Thickness-dependent current-voltage curves of Bi 2 SiO 5 nanoplates measured by C-AFM, showing a high breakdown field strength of 9.4 MV/cm (8.2 nm). Full size image An ideal gate dielectric also needs a large band gap to inhibit the current leakage. Here, vertically grown Bi 2 SiO 5 nanoflakes were directly transferred onto the polished quartz substrate by mechanical pressing for the ultraviolet-visible (UV-vis) absorption measurements. As shown in Fig. 2d , the optical band gap of CVD-grown Bi 2 SiO 5 can be extracted as ~3.80 eV by Tauc’s law, which is consistent with the theoretical value (3.79 eV, Fig. 1b ). To illustrate the metrics of Bi 2 SiO 5 as a gate dielectric, the relationship between band gap and dielectric constant of representative gate dielectrics in literature was plotted in Fig. 2e , clearly indicating the coexistence of high dielectric constant and large band gap in Bi 2 SiO 5 . Moreover, we evaluated the breakdown field strength ( E bd ) of the Bi 2 SiO 5 nanoplates by conductive atomic force microscope (C-AFM) measurements on p ++ Si. As shown in Fig. 2f , the CVD-grown Bi 2 SiO 5 showed thickness-dependent breakdown field strength ranging from 7.2 (13.5 nm) to 9.4 (8.2 nm) MV cm −1 , which is close to that of dielectrics in the silicon industry such as Al 2 O 3 [49] and HfO 2 [50] but owns higher dielectric constant. We should emphasize that the C-AFM is a very local and microscopic tool to measure the breakdown voltage of a dielectric insulator, which may be not the same as the global one determined by MIM device. For example, the breakdown experiments based on the MIM devices gave a breakdown field strength of 3~5 MV/cm instead while varying the thickness of Bi 2 SiO 5 from 10.1 to 21.4 nm (Supplementary Fig. 13 ). The features of easy-to-transfer, ultra-flat surface, high dielectric constant, large band gap, and breakdown field strength make Bi 2 SiO 5 highly competitive as gate dielectrics and high- κ substrates for dielectric screening. Here, we combine Bi 2 SiO 5 with mechanically exfoliated few-layer MoS 2 to construct Bi 2 SiO 5 /MoS 2 FETs for demonstrating its advantages as back-gate dielectrics (Fig. 3 ), dielectric screening substrate (Fig. 4 ) and top-gate dielectrics (Fig. 5 ). Fig. 3: MoS 2 Hall-bar device with the vertically grown ultrathin Bi 2 SiO 5 nanoflake as the high- κ back-gate dielectrics. a OM image of an as-fabricated MoS 2 (~2.7 nm) Hall-bar device on SiO x /Si substrate, in which a thin flake of Bi 2 SiO 5 (~22 nm) and multi-layer graphene were adopted as gate dielectric and back-gate electrode, respectively. b Hall resistance ( R xy ) as a function of magnetic field ( B ) under various gate voltages ( V g ) from 0 to 2 V at 300 K. c The extracted V g -dependent sheet carrier density ( n 2D ), in which a high dielectric constant ( ε r ) of ~36 was derived by linear fitting. The Error bars are based on the standard deviations of slope fitting on R xy - B curves. d Longitudinal resistance ( R xx ) as a function of temperature ( T ) under different V g from 0.4 to 2.0 V, showing a gate-induced insulator-to-metal transition. e Two-probe transfer curves of the back-gated MoS 2 /Bi 2 SiO 5 field-effect transistor (FET) measured by defining the probes of 1 and 4 as source and drain terminals, showing I on / I off > 10 8 , SS ~ 64 mV/decade. The inset shows a small hysteresis of ~15 mV. The extracted two-terminal field-effect mobility of the device is 18.6 cm 2 V −1 s −1 . f The corresponding output curves measured in a V g range from 2 to −2 V. Full size image Fig. 4: Dielectric screening and mobility enhancement effects of CVD-grown Bi 2 SiO 5 nanoflakes as the high- κ substrates. a Schematic illustration and OM image of back-gate MoS 2 four-probe FETs device. b Linear output curves ( I ds – V ds ) of MoS 2 FETs on Bi 2 SiO 5 (left) and on SiO 2 substrate (right) measured at 300 K. c The 4-probe transfer curves of MoS 2 FETs measured at different temperatures (5~300 K) on Bi 2 SiO 5 (left) and SiO 2 (right) substrates, respectively. d The extracted temperature-dependent 4-probe FET mobility ( μ FET,4-probe ) of MoS 2 on Bi 2 SiO 5 (red) and SiO 2 (blue) substrates. Full size image Fig. 5: Hysteresis-free MoS 2 FETs and low-power NMOS inverters using Bi 2 SiO 5 as high- κ top-gate dielectrics. a Schematic illustration of the top-gated MoS 2 FETs on SiO 2 /Si substrate with Bi 2 SiO 5 as the top-gate dielectric. b Typical dual-sweep transfer curves of the MoS 2 /Bi 2 SiO 5 FET measured under different V ds from 0.05 to 1 V, showing an ideal SS value of ~62 mV/decade and ignorable gate hysteresis. The Insert is the OM image of a fabricated MoS 2 FET with Bi 2 SiO 5 as the gate dielectric. c Corresponding output characteristics ( I ds – V ds curves) of the device measured by varying the V g from 0.5 to −0.6 V with a 0.1 V step. d Extracted SS value versus I ds characteristics of the device in b , showing a low SS value (<70 mV/decade) for a wide I ds range. e Dual gated transfer curves of the MoS 2 / Bi 2 SiO 5 FET under different back-gate voltages ( V BG ) from 5 to 0 V. f The extracted threshold voltage V th from e as a function of V BG . The linear fitting yields a slope of −0.0097 and a high dielectric constant of ~32.3. g The thickness-dependent dielectric constant of Bi 2 SiO 5 extracted by dual-gate measurement on Bi 2 SiO 5 /MoS 2 /SiO 2 /Si FET. The dotted curve is a visual guide. h Transfer curves of the MoS 2 FETs with different thickness Bi 2 SiO 5 as the top-gate dielectrics, showing a trend of smaller V th for thinner Bi 2 SiO 5 thickness. The V ds is 0.5 V , and no V BG is applied. i Measured output voltage ( V out ) and gain as a function of input voltage ( V in ) of an NMOS inverter based on two MoS 2 / Bi 2 SiO 5 FETs under different supply voltage ( V dd ) from 2 V to 0.5 V. Full size image Vertically grown Bi 2 SiO 5 as back-gate dielectric The small contact area and weak interaction between the vertically grown Bi 2 SiO 5 and the mica substrate make it compatible with the well-developed aligned transfer method (For details, see Supplementary Fig. 14 ) [19] , [20] , allowing us to fabricate complex vdWs heterojunction devices by layer-by-layer stacking. 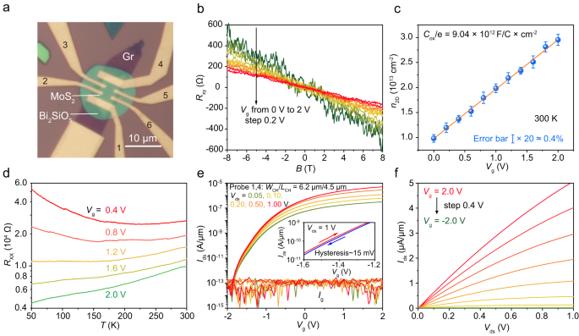Fig. 3: MoS2Hall-bar device with the vertically grown ultrathin Bi2SiO5nanoflake as the high-κback-gate dielectrics. aOM image of an as-fabricated MoS2(~2.7 nm) Hall-bar device on SiOx/Si substrate, in which a thin flake of Bi2SiO5(~22 nm) and multi-layer graphene were adopted as gate dielectric and back-gate electrode, respectively.bHall resistance (Rxy) as a function of magnetic field (B) under various gate voltages (Vg) from 0 to 2 V at 300 K.cThe extractedVg-dependent sheet carrier density (n2D), in which a high dielectric constant (εr) of ~36 was derived by linear fitting. The Error bars are based on the standard deviations of slope fitting onRxy-Bcurves.dLongitudinal resistance (Rxx) as a function of temperature (T) under differentVgfrom 0.4 to 2.0 V, showing a gate-induced insulator-to-metal transition.eTwo-probe transfer curves of the back-gated MoS2/Bi2SiO5field-effect transistor (FET) measured by defining the probes of 1 and 4 as source and drain terminals, showingIon/Ioff> 108,SS~ 64 mV/decade. The inset shows a small hysteresis of ~15 mV. The extracted two-terminal field-effect mobility of the device is 18.6 cm2V−1s−1.fThe corresponding output curves measured in aVgrange from 2 to −2 V. Figure 3a showed the OM image of an as-fabricated MoS 2 Hall-bar device using Bi 2 SiO 5 as the back-gate dielectric and multi-layer graphene as a back-gate electrode. Gated Hall measurement is a powerful tool to get a series of key parameters, such as the dielectric constant of the gate dielectric, carrier density, and Hall mobility of the channel semiconductor. Besides, it also enables us to get the transfer and output characteristics by defining two out of six electrodes as source and drain. Figure 3b showed Hall resistance ( R xy ) as a function of magnetic field ( B ) under different gate voltages ( V g ) at room temperature, from which we can extract the V g -dependent sheet carrier densities ( n 2D ). By linear fitting the curve of n 2D - V g (Fig. 3c ), the estimated slope equals the C ox /e, where C ox is capacitance density and e is the elementary charge. The C ox for a 22-nm-thick Bi 2 SiO 5 can be as high as 1.45 μF/cm 2 , suggesting a very high dielectric constant ( ɛ r ~ 36), which is consistent with the value extracted by C – V measurements in a reasonable accuracy. On the other hand, very large capacitance density suggests that we can greatly regulate the carrier density and electrical behavior of the MoS 2 semiconductor. As confirmed by the room-temperature Hall measurements (Fig. 3c ), a very high carrier density of 1.83 × 10 13 cm −2 can be doped into the channel by applying a V g of 2 V on Bi 2 SiO 5 dielectrics. To this end, the temperature-dependent longitudinal resistance ( R xx - T ) behavior of MoS 2 can be greatly regulated from insulating to metallic one when sweeping the V g from 0.4 to 2 V (Fig. 3d ), indicating the great potential of Bi 2 SiO 5 dielectric as a powerful tool for physical state regulation. To examine whether ultrathin Bi 2 SiO 5 can serve as excellent back-gate dielectrics of a FET, we define the electrodes #1, #4 and graphene as source, drain, and gate electrodes, respectively. The dual-sweep transfer curves of MoS 2 /Bi 2 SiO 5 /Gr FET were presented in Fig. 3e , showing a large I on / I off of >10 8 , and a small SS value of ~64 mV/decade. Considering the relatively complex device fabrication process (Supplementary Fig. 14 ), chemical residuals will inevitably remain at the interfaces between the graphene, Bi 2 SiO 5 and MoS 2 , which are detrimental to the device performance. Nevertheless, the FET still exhibited small hysteresis of ~15 mV, which is comparable to the value obtained after interface optimization [51] . Thanks to the Ohmic contact formed by In/Au electrodes (Fig. 3f ), two-terminal field-effect mobility of the device can be as high as 18.6 cm 2 V −1 s −1 by linear fitting the transfer curve, which is comparable to the Hall mobility measured at room temperature (23.7 cm 2 V −1 s −1 at V g = 2 V, Supplementary Fig. 15 ). Notably, Bi 2 SiO 5 was also verified as an excellent gate insulator while shrinking the channel length of MoS 2 FETs down to 100 nm and even 30 nm (Supplementary Figs. 16 , 17 ). Vertically grown Bi 2 SiO 5 as high- κ screening layer Dangling bonds on SiO 2 /Si substrate usually act as the scattering sites of Coulomb impurities (CI) to decrease the mobility of a semiconductor [52] , [53] , [54] . Theoretically speaking, using an h -BN-like high- κ substrate free of dangling bonds can effectively enhance its mobility due to reduced CI scatterings and excellent dielectric screening. 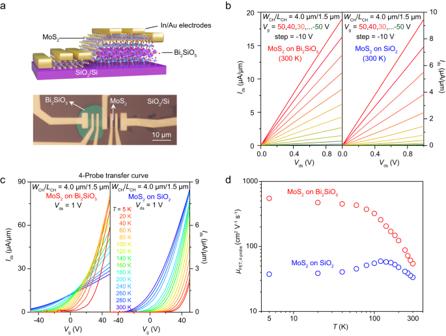Fig. 4: Dielectric screening and mobility enhancement effects of CVD-grown Bi2SiO5nanoflakes as the high-κsubstrates. aSchematic illustration and OM image of back-gate MoS2four-probe FETs device.bLinear output curves (Ids–Vds) of MoS2FETs on Bi2SiO5(left) and on SiO2substrate (right) measured at 300 K.cThe 4-probe transfer curves of MoS2FETs measured at different temperatures (5~300 K) on Bi2SiO5(left) and SiO2(right) substrates, respectively.dThe extracted temperature-dependent 4-probe FET mobility (μFET,4-probe) of MoS2on Bi2SiO5(red) and SiO2(blue) substrates. Figure 4a shows the scheme and OM image of as-fabricated 4-probe MoS 2 FETs on top of Bi 2 SiO 5 and SiO 2 /Si substrates. To avoid the influence of sample quality variation, one MoS 2 sample (4.3 nm) was simultaneously placed on Bi 2 SiO 5 (31.9 nm) and SiO 2 substrates for comparison. As demonstrated in Fig. 4b , the V g -dependent two-probe I – V curves (output characteristics) were measured at 300 K, showing a linear behavior over a large voltage window, confirming the Ohmic contact formed by In/Au electrodes. It’s worth noting that the on-state current ( I on ) of MoS 2 on Bi 2 SiO 5 is about twice as the one on SiO 2 , suggesting a higher mobility of MoS 2 on Bi 2 SiO 5 substrate. To illuminate the influence of contact resistance, 4-probe transfer curves were measured among a temperature range of 5~300 K (Fig. 4c ). By linear fitting the transfer curves, we can extract the 4-probe FET mobility ( μ FET,4-probe ) as a function of temperature (Fig. 4d ). Among the whole temperature range of 300~5 K, the carrier mobility of MoS 2 on Bi 2 SiO 5 is significantly higher than that on SiO 2 /Si substrate, which can be further confirmed by plotting the I ds as a function of a normalized V g by threshold voltage ( V g - V th , Supplementary Fig. 18 ). Particularly, the mobility of MoS 2 on Bi 2 SiO 5 at 5 K is as high as 549.3 cm 2 V −1 s −1 , which is almost fifteen times higher than the value of MoS 2 on SiO 2 /Si (~37.4 cm 2 V −1 s −1 ). Moreover, the carrier mobility of MoS 2 on Bi 2 SiO 5 and SiO 2 /Si showed totally different temperature dependence. For MoS 2 /Bi 2 SiO 5 , its carrier mobility increased monotonously upon cooling down, suggesting the phonon scattering dominated the whole transport events even at low temperature. In contrast, the carrier mobility of MoS 2 on SiO 2 /Si substrate increased first while cooling down to ~150 K, but gradually decreased upon further cooling. This T -dependent mobility can be well explained by enhanced charge impurities scattering at low temperature in MoS 2 /SiO 2 interface. In a word, using Bi 2 SiO 5 as a substrate greatly improve the performance of the MoS 2 FET to get a higher mobility, which can be attributed to the suppressed CI scatterings in the high- κ surroundings and ideal dielectric/semiconductor interface. Vertically grown Bi 2 SiO 5 as the top-gate dielectric Top-gate FET is a widely used device configuration in practical applications. In this part, we fabricated Bi 2 SiO 5 /MoS 2 top-gate FETs to prove the feasibility of Bi 2 SiO 5 as top-gate dielectric layer in hysteresis-free low-power transistors (Supplementary Fig. 19 ). As shown in Fig. 5a , the Bi 2 SiO 5 /MoS 2 top-gate FET was placed on the SiO 2 /Si substrate, which can also serve as the back-gate dielectric and electrode when necessary. 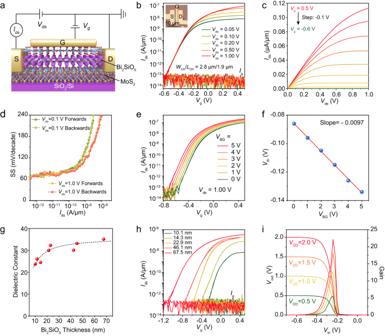Fig. 5: Hysteresis-free MoS2FETs and low-power NMOS inverters using Bi2SiO5as high-κtop-gate dielectrics. aSchematic illustration of the top-gated MoS2FETs on SiO2/Si substrate with Bi2SiO5as the top-gate dielectric.bTypical dual-sweep transfer curves of the MoS2/Bi2SiO5FET measured under differentVdsfrom 0.05 to 1 V, showing an idealSSvalue of ~62 mV/decade and ignorable gate hysteresis. The Insert is the OM image of a fabricated MoS2FET with Bi2SiO5as the gate dielectric.cCorresponding output characteristics (Ids–Vdscurves) of the device measured by varying theVgfrom 0.5 to −0.6 V with a 0.1 V step.dExtractedSSvalue versusIdscharacteristics of the device inb, showing a low SS value (<70 mV/decade) for a wideIdsrange.eDual gated transfer curves of the MoS2/ Bi2SiO5FET under different back-gate voltages (VBG) from 5 to 0 V.fThe extracted threshold voltageVthfromeas a function ofVBG. The linear fitting yields a slope of −0.0097 and a high dielectric constant of ~32.3.gThe thickness-dependent dielectric constant of Bi2SiO5extracted by dual-gate measurement on Bi2SiO5/MoS2/SiO2/Si FET. The dotted curve is a visual guide.hTransfer curves of the MoS2FETs with different thickness Bi2SiO5as the top-gate dielectrics, showing a trend of smallerVthfor thinner Bi2SiO5thickness. TheVdsis 0.5V, and noVBGis applied.iMeasured output voltage (Vout) and gain as a function of input voltage (Vin) of an NMOS inverter based on two MoS2/ Bi2SiO5FETs under different supply voltage (Vdd) from 2Vto 0.5 V. Figure 5b showed the typical dual-sweep transfer curves of a 22.9-nm-thick Bi 2 SiO 5 -based MoS 2 FET measured under different V ds from 0.05 to 1 V. Owing to the excellent gate tunability, the transistor can be effectively turned on and off by applying a V g within the range of −0.6~0.5 V, showing a large I on / I off of >10 6 and a low gate leakage current of 10 −13 A (approaching the detection limit). Furthermore, the ideal SS value (~62 mV/decade), ignorable gate hysteresis (~3 mV), and low drain-induced barrier lowering (DIBL, ~5 mV/V) suggest the perfect interface was formed at MoS 2 /Bi 2 SiO 5 interface (Supplementary Fig. 20 ). The MoS 2 transistor showed a linear I ds - V ds curve at low V ds region, then gradually saturated at high V ds region (Fig. 5c ). Particularly, the SS remains low (<70 mV/decade) for different I ds of several orders of magnitude for both forward and reverse top-gate sweeping (Fig. 5d ). More importantly, the top-gate Bi 2 SiO 5 /MoS 2 short-channel FET, whose channel length was defined by the gap distance between two graphene electrodes (~180 nm), still showed a small DIBL value of ~22 mV/V and SS value of ~79 mV/decade (Supplementary Fig. 21 ). One step further, nearly hysteresis-free transfer curves were preserved in a dual-gate FET configuration, in which a back-gate voltage ( V BG ) was employed to modulate the threshold voltage ( V th ) of the device. As a result, the top-gate transfer curves gradually shifted as the V BG varied from 5 to 0 V (Fig. 5e and Supplementary Fig. 22 ). By linear fitting the V th as a function of V BG , we can extract a slope of −0.0097, which equals to the ratio of the bottom-gate to top-gate capacitance, namely C (SiO 2 )/ C (Bi 2 SiO 5 ), when the parallel-plate capacitor model is assumed for both top and bottom gates [16] , [55] . For a 285 nm SiO 2 dielectric ( ɛ r = 3.9), its capacitance can be calculated as 0.0121 μF/cm 2 . In this case, the capacitance and dielectric constant for a 22.9-nm-thick Bi 2 SiO 5 were derived as 1.25 μF/cm 2 and 32.3, both of which matched well with the value obtained by C – V (Fig. 2a ) and gated Hall measurements (Fig. 3c ). Next, the interface trap density D it was extracted based on the following equation: [15] 
    SS=ln(10)k_BT/q(1+qD_it/C_ox)
 (1) where SS is the subthreshold swing, k B is Boltzmann constant, T is absolute temperature, q is the elementary charge, C ox is the gate capacitance obtained from MOS capacitance measurements. As a result, a low D it value of 2.88 × 10 11 cm −2 /eV was extracted, verifying the high quality of the vdWs interface. Moreover, the dielectric constant of Bi 2 SiO 5 , extracted by dual-gate transfer measurements, also showed similar thickness dependence with the C – V results (Fig. 5g ). Figure 5h plotted the dual-sweep transfer curves of MoS 2 FETs with different Bi 2 SiO 5 thicknesses (10.1~67.5 nm). Apparently, smaller V g is needed to switch the transistor on and off when a thinner Bi 2 SiO 5 dielectric is used. We should emphasize that the EOT value for a 10.1 nm Bi 2 SiO 5 is as small as 1.3 nm, but its gate leakage current is still on the order of 10 −13 A, signifying substantial room space for further scaling of EOT and great potential applications in low-power devices. The I on of MoS 2 FETs in Fig. 5h seems to decrease with decreasing the thickness of Bi 2 SiO 5 , which may originate from the contact issues existing in the MoS 2 FETs with the thin Bi 2 SiO 5 as gate insulators. However, we should emphasize that, the I on of ultrathin Bi 2 SiO 5 -gated MoS 2 FETs can be greatly improved by optimizing the device fabrication process. As shown in Supplementary Figs. S23 – 25 , the I on of another 10-nm-thick Bi 2 SiO 5 -gated MoS 2 can be similar to the value of the thick Bi 2 SiO 5 -gated FETs (0.11 μA/μm, Fig. 5b ). It is worth noting that the I on is greatly limited by the remaining ungated channel in the top-gate device configuration. Additionally, as confirmed by the dual-sweep transfer curves, a nearly ideal SS value and a low normalized gate hysteresis can indeed be obtained in the Bi 2 SiO 5 gated MoS 2 FET. The low operating voltage is essential to fabricate low-power logic circuits. As demonstrated in Fig. 5i , we used two n-type transistors as the load and driver terminal to construct 2D inverter with a high voltage gain of 22.0. The inverter can demonstrate the logic state 0 and 1 within ±0.5 V, showing a low dynamic power consumption of <0.7 nW (Supplementary Fig. 26 ). In summary, our work achieved the direct CVD growth of ultrathin free-standing high -k single-crystalline dielectrics, which is much more efficient than traditional mechanical exfoliation. The vertically grown Bi 2 SiO 5 2D crystals present the metrics for a gate dielectric, as evidenced by the coexistence of high dielectric constant, large band gap, high breakdown field strength, as well as the characteristic of easy transfer by facile polymer-free mechanical pressing. These features make Bi 2 SiO 5 attractive as an inert vdWs substrate superior to h -BN for exploring exotic transport properties under reduced interfacial scatterings and stronger gate control, as well as for fabricating hysteresis-free 2D transistors with scaled supply voltage. CVD growth of ultrathin Bi 2 SiO 5 nanoplates on mica substrate 2D Bi 2 SiO 5 crystals were synthesized inside a homemade CVD system equipped with a single heating zone tube furnace and 30 mm diameter quartz tube. Typically, the BiF 3 powders (purity 99.999%, Macklin) were placed in an empty quartz boat or on top of the SiO 2 powders located in the heating center, and the freshly cleaved fluorophlogopite mica substrates were placed above the quartz boat. The heating temperature of the source was 600–750 °C and the growth time was 20 min. The 50 s.c.c.m Ar and 5 s.c.c.m mixed Ar/O 2 (1‰) gas were introduced into the CVD system as carrier gas. The system pressure was kept constant as 760 Torr during the whole growth process. Characterization of CVD-grown ultrathin Bi 2 SiO 5 single-crystalline dielectric The morphologies of as-synthesized in-plane and free-standing 2D Bi 2 SiO 5 nanoplates were characterized by optical microscopy (Olympus BX53), scanning electron microscopy (SEM, JSM-7800F) and atomic force microscope (AFM, Bruker dimension icon). With a polymer-free method of mechanical pressing, vertically grown Bi 2 SiO 5 nanoflakes were transferred onto Cu grid, glass, and optical quartz substrates to perform the characterizations of transmission electron microscopy (TEM, JEM 2800), X-ray diffraction (XRD, Rigaku Smart Lab 30 KW) and absorption spectrum (SHIMADZU, UV-2600), respectively. The Raman spectroscopy was measured on WITec alpha300R with a laser of 532 nm. The cross-sectional TEM samples of in-plane and vertically grown Bi 2 SiO 5 nanoflakes were both prepared by using a focused ion/electron dual beam system (FEI, Helios 5 CX). All cross-sectional scanning transmission electron microscopy (STEM) imaging was obtained on an aberration-corrected TEM operating at 300 kV (FEI Titan cubed Themis G2 300). The breakdown field strength of Bi 2 SiO 5 was measured with the C-AFM module of Bruker Dimension Icon. First-principles calculations The structural relaxation of Bi 2 SiO 5 is performed within the framework of density function theory (DFT) using the projector augmented wave pseudopotential and the Perdew–Burke–Ernzerhof exchange-correlation functional as implemented in the VASP. The energy cutoff for the plane-wave expansion is set to 500 eV, and a Monkhorst–Pack k-mesh of 3 × 9 × 9 is used in the Brillouin zone. The energy convergence threshold is 10 −6 eV and the force 10 −3 eV Å −1 in the structural optimization. In order to overcome the underestimation of energy gap from the generalized gradient approximation (GGA), we use the method of modified Becke–Johnson potential (mBJ) to calculate the electronic structure. Device fabrication To illuminate the possible capacitance coupling, the Bi 2 SiO 5 -based metal-insulator-metal (MIM) capacitors were fabricated on quartz substrates rather than SiO 2 /Si substrates. First, the thick graphite was exfoliated onto the quartz substrate as bottom electrodes for its ultrasmooth surface. Next, the vertically grown Bi 2 SiO 5 nanoflakes were directly picked up from the mica substrate by a polypropylene carbonate/polydimethylsiloxane (PPC/PDMS) stamp, followed by aligned transfer onto the specific graphite bottom electrode by a high-precision transfer platform. Subsequently, the standard electron-beam lithography (EBL) process and thermal evaporation were used to pattern the top electrodes ((In/Au, 5/40 nm). For fabricating the back-gated MoS 2 Hall-bar device using graphite as bottom electrodes, the detailed process was listed as follows. First, SiO 2 /Si substrates (285 nm SiO 2 ) were pretreated with O 2 plasma (Diener Pico plasma cleaner) for 5 min at a power of 50 W. Next, few-layer MoS 2 and graphite were exfoliated onto different SiO 2 /Si substrates. With the help of the PPC/PDMS stamp and high-precision transfer platform, the free-standing Bi 2 SiO 5 and MoS 2 nanoflakes were sequentially stacked on top of the graphite. The six-terminal electrode legs for the Hall-bar and the bottom metal electrodes were simultaneously written by one-step EBL and following thermal metal deposition (In/Au, 5/40 nm). The device fabrication process of 4-terminal MoS 2 FET includes the following parts: (1) transfer the Bi 2 SiO 5 onto SiO 2 /Si substrate by mechanical pressing; (2) place part of the few-layer MoS 2 on top of the Bi 2 SiO 5 nanosheet; (3) EBL and metal deposition (In/Au, 5/40 nm). For the top-gated MoS 2 device, few-layer MoS 2 nanosheets were exfoliated onto SiO 2 /Si substrate, followed by stacking Bi 2 SiO 5 nanoflakes in the middle of the MoS 2 nanosheets as the gate dielectrics. The source, drain, and top-gate electrodes of MoS 2 FETs were patterned together with one-step EBL process and thermal metal evaporation (In/Au, 5/40 nm). Electrical transport measurements 2-probe electrical properties of the back-gate and top-gate MoS 2 FETs, including the Figs. 3 e, f, 4 b, 5b, c, e, h , were carried out by a semiconductor analyzer (FS-Pro) in a shielded vacuum chamber (<0.1 Torr) at room temperature, whose noise level is ~1 × 10 −13 A within the voltage range of ±2 V. The 4-probe transfer curves and gated 4-probe measurements (such as gated R xx - T and Hall data), including Figs. 3 b, d, 4c , were carried out in a Physical Properties Measurement Systems (PPMS-9T, Quantum Design) equipped with a homemade electrical measurement system, which is composed of 2 Keithley 2400, and 2 Keithley 2182 A nanovoltmeter and has a noise level of ~10 −10 A within the voltage range of ± 2 V. The C – V and C – f measurements were carried out on a FS336 LCR Meter.